Mutants of Cre recombinase with improved accuracy Despite rapid advances in genome engineering technologies, inserting genes into precise locations in the human genome remains an outstanding problem. It has been suggested that site-specific recombinases can be adapted towards use as transgene delivery vectors. The specificity of recombinases can be altered either with directed evolution or via fusions to modular DNA-binding domains. Unfortunately, both wild-type and altered variants often have detectable activities at off-target sites. Here we use bacterial selections to identify mutations in the dimerization surface of Cre recombinase (R32V, R32M and 303GVSdup) that improve the accuracy of recombination. The mutants are functional in bacteria, in human cells and in vitro (except for 303GVSdup, which we did not purify), and have improved selectivity against both model off-target sites and the entire E. coli genome. We propose that destabilizing binding cooperativity may be a general strategy for improving the accuracy of dimeric DNA-binding proteins. Safe delivery of transgenes into the human genome remains an open problem of critical importance to clinical genetics. Many existing technologies have major limitations. For instance, retroviruses, lentiviruses and transposons integrate non-specifically and can therefore cause cancer by mutagenesis [1] , [2] . Transgenes can also be integrated using the endogenous homologous repair pathways, although this process must be stimulated by generating double-stranded breaks at the target site using programmable nuclease technologies, such as meganucleases [3] , zinc finger nucleases [4] , TALE nucleases [5] , [6] or the RNA-guided Cas9 protein [7] , [8] . This technique is limited by the fact that homologous recombination in humans is less efficient than the competing mutagenic non-homologous end-joining pathway [9] , [10] . Site-specific recombinases, which catalyse recombination at precise sites, have properties that make them promising candidates for use as safe gene-delivery vectors. For instance, many do not require host-encoded factors [11] . In addition, the size of the integrated cassette is less restricted than for other methods. Recombinases’ specificities can be altered either by direction evolution or by fusion to modular DNA-binding domains [12] , [13] , [14] , [15] , [16] , [17] , [18] , [19] , [20] . Unfortunately, many reprogrammed variants are promiscuous in their activity. This problem is not restricted to artificial variants, as activity at off-target human genomic loci has been reported for some wild-type (WT) recombinases [21] , [22] , [23] , [24] . If recombinases are to be used as gene-delivery vectors, it is imperative to identify ways to enhance their accuracy. The accuracy of DNA-binding proteins can be altered by varying the ratio of specific to non-specific DNA–protein interactions [25] . Although powerful, this approach can be inconvenient if the goal is to generate variants of a protein with different specificities: a specificity change alters the DNA–protein interaction, requiring re-optimization of accuracy. Therefore, there is a need for methods to systematically enhance accuracy without changing the DNA–protein interface. In this work, we attempt to discern such principles using Cre recombinase of the phage P1 as a model system. Cre catalyses a reversible, directional recombination between two 34 bp loxP sites that consist of a pair of 13 bp inverted repeats flanking an 8 bp asymmetrical spacer [26] , [27] , [28] . Mutagenic studies of loxP have shown that many mutations have non-catastrophic effects on recombination efficiency [29] , [30] , [31] . Using a theoretical model, we predict that reducing the cooperativity of binding should increase accuracy. We mutagenize a region involved in the formation of Cre dimers and perform bacterial selections for functional and accurate mutants. We isolate three mutants, all of which were able to recombine loxP sites with high efficiency and exhibited improved accuracy with respect to both model off-target sites and the entire Escherichia coli genome. A theoretical model of DNA-binding accuracy Under the currently accepted mechanism of Cre recombination, the binding of a Cre monomer to one half of a loxP site is followed by the formation of an asymmetrical homodimer when a second Cre molecule binds to the other half of loxP . Next, the two loxP -bound dimers associate to form a tetramer, and recombination proceeds via a Holiday Junction intermediate [28] . We reasoned that the formation of the dimer of dimers is not site specific in the sense that it involves no new DNA-binding events, leading us to conclude that the precision of dimer formation determines the accuracy of recombination. Assuming that the protein–protein affinity is negligible in the absence of DNA, dimer formation on target sites is described with: where P is the unbound protein monomer, D is the full DNA-binding site, K is the affinity of each monomer for half of the binding site and K dim is the affinity of the protein dimer for the full binding site. If it is assumed that the cooperative energy is sequence-independent then K dim = KK coop , where K coop is the protein–protein affinity. A competing set of binding events occurs between off-target DNA and the protein: where D OT is the off-target DNA concentration and K OT is the affinity of the protein for off-target DNA. Accuracy can be defined as the ratio of on-target protein dimers to off-target protein dimers: The free DNA concentration [ D ] is related to the total DNA concentrations [ D total ] via: An analogous expression relates [ D OT ] and [ D OT,total ]. Equation (5) can be expressed in terms of total DNA concentrations: To model accuracy of Cre in E. coli , we used the in vitro affinity coefficients K of 1.5 × 10 8 M −1 and a K coop of 1.7 × 10 3 M −1 , with both values obtained from previous in vitro measurements [32] . We assumed that K / K OT =10 4 , which is in the same order of magnitude as the experimentally determined K / K OT of Eco RV and Bam HI [33] . Assuming a single target site in an E. coli cell of a 0.5 μm radius gives a [ D total ] of 3.2 × 10 −9 M. If off-target sites exist at 1 bp windows along both strands of the 4.6 Mbp E. coli genome, then [ D OT,total ] is ~3.2 × 10 −9 M bp −1 × 9.2 × 10 6 bp=2.9 × 10 −2 M. This value of [ D OT,total ] may be an overestimate owing to competitive binding of other DNA-associated proteins to the genome. We plotted the predicted accuracy of dimer formation as a function of total protein concentration for both WT Cre and for mutants with reduced cooperativity ( Fig. 1 ). The model predicts that accuracy increases with both a reduction in cooperativity and a decrease in protein expression levels. This is an intuitive result, because accuracy should increase as the two monomer binding events become more independent from each other. We conclude that although a reduction in cooperative binding will affect both target and off-target binding, off-target binding will be destabilized to a greater degree. 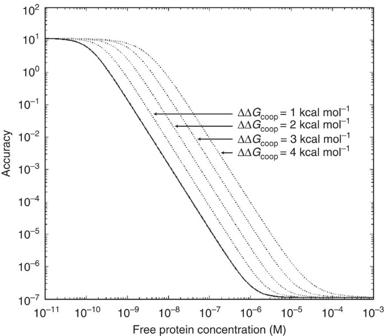Figure 1: Model predicting an increase in Cre recombinase dimer binding accuracy as cooperativity decreases. The solid line indicates the accuracy predicted for WT Cre, whereas the dashed lines correspond to the expected accuracy of mutants in which the cooperativity has been reduced by the indicated amount. Figure 1: Model predicting an increase in Cre recombinase dimer binding accuracy as cooperativity decreases. The solid line indicates the accuracy predicted for WT Cre, whereas the dashed lines correspond to the expected accuracy of mutants in which the cooperativity has been reduced by the indicated amount. Full size image Identifying candidate mutations using bacterial selection Our theoretical model predicted that accuracy could be improved by decreasing the cooperative binding moment. We therefore targeted our mutagenesis towards a domain directly involved in the dimer interaction but distant from the Cre–DNA interaction: the α-helix closest to the amino terminus [34] . To find mutations that improve accuracy while maintaining proper function with respect to loxP , we performed two rounds of bacterial selection. The first round was designed to identify functional mutants, whereas the second round selected accurate mutants. To select functional mutants, we used a resistance marker flanked by loxP sites in an inverted orientation relative to each other. The reading frame was inverted with respect to the promoter, such that Cre-mediated inversion would result in gain of antibiotic resistance. An out-of-frame toxic ccdB was used to apply a selective pressure against inaccurate recombination reactions that produced frameshifts ( Fig. 2a ). To minimize false negatives due to reversal of the inversion, we placed the selection cassette on a high copy plasmid. The selection resulted in the recovery of 1,690 library-transformed colonies, which corresponds to 38% of the total transformation efficiency. The library produced fewer clones than the positive WT control, suggesting that the selection is functional ( Fig. 2b ). 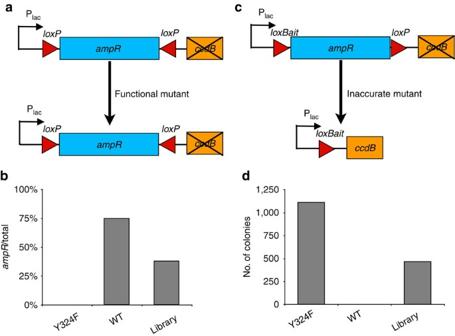Figure 2: Selecting functional and accurate Cre variants. (a) The substrate used to select for functional variants; proper recombination would place the ampicillin resistance gene (ampR) under the lac promoter (Plac) conferring resistance. TheccdBgene is crossed out to indicate that it’s out of frame with respect to the ampR start codon. (b) Ratio of ampicillin-resistant colonies to total colonies isolated following the positive selection. (c) The substrate used to select for accurate variants—recombination ofloxPandloxBaitsites would result in loss of ampicillin resistance and would place the toxicccdBgene in frame with the promoter. (d) Number of ampicillin-resistant colonies recovered from the negative selection. Figure 2: Selecting functional and accurate Cre variants. ( a ) The substrate used to select for functional variants; proper recombination would place the ampicillin resistance gene ( ampR ) under the lac promoter (P lac ) conferring resistance. The ccdB gene is crossed out to indicate that it’s out of frame with respect to the ampR start codon. ( b ) Ratio of ampicillin-resistant colonies to total colonies isolated following the positive selection. ( c ) The substrate used to select for accurate variants—recombination of loxP and loxBait sites would result in loss of ampicillin resistance and would place the toxic ccdB gene in frame with the promoter. ( d ) Number of ampicillin-resistant colonies recovered from the negative selection. Full size image To identify accurate constructs, we first found an off-target site to serve as bait in the negative selection. To achieve a high selective pressure, we wanted a bait sequence that would be recombined with a high efficiency. At the same time, we wanted to select for improved accuracy across the entire protein–DNA interaction and, therefore, we wanted a bait sequence with little similarity to loxP . We found such a site by performing a selection for pseudo- loxP sites and characterizing their in vitro recombination efficiency. The site, which we named loxBait , is recombined with 37% the efficiency of loxP , despite differences in 9 out of 13 bases within a single inverted repeat ( Fig. 3a,b ). 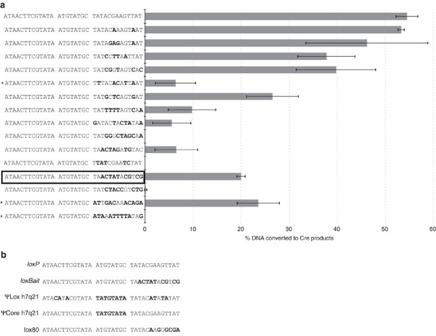Figure 3:Activity and nomenclature of pseudo-loxPsites. (a) Linear fragments withloxPon one end and the indicated sites on the other were treated with Cre and the products were quantified on an agarose gel. All new bands were counted towards the recombination efficiency. No recombination was observed for any of the sites in the absence of Cre. Bolded positions correspond to differences fromloxP. Sites are listed in order of similarity withloxP. Asterisks mark sequences generated randomly; all others were obtained from a selection for functional pseudo-loxPsites. The box indicatesloxBait. (b) The names and sequences of recombination sites used in this study. Positions that are different fromloxPare shown in bold. Error bars correspond to 95% CI (n=two to three experimental replicates). Figure 3: Activity and nomenclature of pseudo- loxP sites. ( a ) Linear fragments with loxP on one end and the indicated sites on the other were treated with Cre and the products were quantified on an agarose gel. All new bands were counted towards the recombination efficiency. No recombination was observed for any of the sites in the absence of Cre. Bolded positions correspond to differences from loxP . Sites are listed in order of similarity with loxP . Asterisks mark sequences generated randomly; all others were obtained from a selection for functional pseudo- loxP sites. The box indicates loxBait . ( b ) The names and sequences of recombination sites used in this study. Positions that are different from loxP are shown in bold. Error bars correspond to 95% CI ( n =two to three experimental replicates). Full size image We performed the counterselection by flanking an in-frame antibiotic resistance marker with loxBait and loxP oriented in the same direction. The toxic ccdB gene was placed at the 3′-end of loxP . Cre-mediated excision would result in both loss of the resistance marker and expression of the toxic gene ( Fig. 2c ). We subjected the expression plasmids recovered from the positive selection to one round of counterselection. In this case, the catalytically inactive mutant, Y324F, served as the control for growth without selection ( Fig. 2d ). We randomly isolated two of the recovered mutants, R32V and R32M, for further characterization. R32 is involved in an intermonomer salt bridge with E69; thus, its disruption in the two mutants can be expected to reduce the protein–protein affinity ( Fig. 4a ). Two WT colonies survived the counterselection, one of which contained a clone with a de novo duplication of residues 303–305 (303GVSdup). This region is a loop that makes close contact to the other monomer in the dimer structure ( Fig. 4b ). 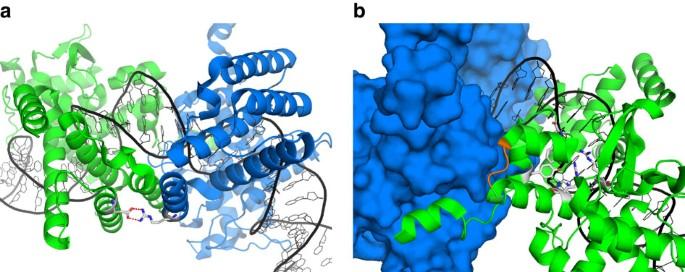Figure 4: Structural context of the isolated mutants. (a) R32V and R32M disrupt a putative salt bridge between two monomers (shown in blue and green) at R32 and E69. The two residues are shown as stick structures coloured by atom identity (blue–N; red–O; gray–C). (b) 303GVSdup duplicated the loop shown in orange. One of the monomers is shown as a space-filling model. The catalytic site residues (R173, H289, R292, W315 and Y324) are shown as stick figures. The crystallographic data was obtained from PDB 3C29. Figure 4: Structural context of the isolated mutants. ( a ) R32V and R32M disrupt a putative salt bridge between two monomers (shown in blue and green) at R32 and E69. The two residues are shown as stick structures coloured by atom identity (blue–N; red–O; gray–C). ( b ) 303GVSdup duplicated the loop shown in orange. One of the monomers is shown as a space-filling model. The catalytic site residues (R173, H289, R292, W315 and Y324) are shown as stick figures. The crystallographic data was obtained from PDB 3C29. Full size image Mutants better discriminate a model off-target site We measured the activity of Cre and the isolated mutants on loxP and ψLox h7q21 , a known human off-target site [21] , using a plasmid-based inversion assay. As in the selections, the proteins were expressed from the P bad promoter. As our theoretical model suggests that greater accuracy is achieved at low protein expression levels, we grew the cells on repressive LB/glucose medium. Indistinguishable results were achieved with growth on LB in the absence of glucose. To test the mutants for improved accuracy, we analysed their ability to recombine a known human pseudo- loxP site ψLox h7q21 and ψCore h7q21 (which consists of inverted repeats from loxP but a spacer that matches ψLox h7q21F ; Fig. 3b ). Following recombination, substrate plasmids were isolated and digested in a way that resulted in the substrate producing a 631-bp band and its inverted product producing a 386-bp band ( Fig. 5a ). Y324F produced only the 631-bp parent product, whereas R32V, R32M and 303GVSdup resulted in both inverted and parental plasmids ( Fig. 5b ). WT unexpectedly produced the 898-bp band that corresponds to a deletion; there were no detectable bands for the inverted and parental forms. We also observed a 1,795-bp band formed when Sca I failed to cut. This product could be ignored for Y324F, R32V, R32M and 303GVSdup, because the cutting efficiency of Sca I should be independent of cassette orientation. However, the 1,795-bp band did need to be taken into account when analysing recombination by WT: we normalized the 898-bp deletion product band to the total amount of DNA in the 898- and 1,795-bp bands ( Fig. 5c,d ). Incomplete Sca I digests also produced a 2,573-bp product that is formed via an intermolecular insertion followed by inversion between recombination sites that originated from different molecules ( Supplementary Fig. S1 ). We excluded this product from our analysis. 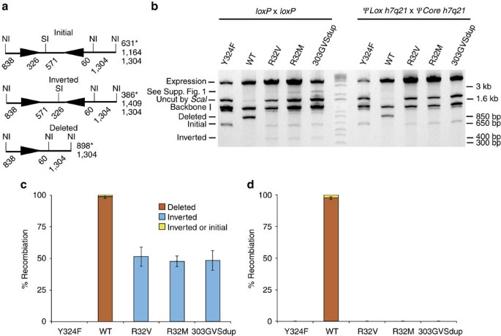Figure 5:In vivorecombination of plasmids by mutants of Cre. (a) Plasmid architecture of the three expected recombination products. Recombination sites are shown as triangles. For simplicity, the map is in linear form, where theNcoI sites at the ends represent a singleNcoI site on the circular plasmids. The numbers under each segment indicate distance in bp (map not drawn to scale). The numbers adjacent to each map are the sizes of the expected digestion products, with the asterisks indicating the product size that is unique to the particular configuration. (b) Digest analysis ofloxP×loxP(left five lanes) andψlox h7q21×ψCore h7q21(right five lanes) recombination. (c,d) Inversion and recombination frequency of (c)loxP×loxPand (d)ψlox h7q21×ψCore h7q21recombination obtained by quantifying band intensities. Error bars correspond to 95% CI (n=two independent experiment). NI,NcoI site; SI,ScaI site. Figure 5: In vivo recombination of plasmids by mutants of Cre. ( a ) Plasmid architecture of the three expected recombination products. Recombination sites are shown as triangles. For simplicity, the map is in linear form, where the Nco I sites at the ends represent a single Nco I site on the circular plasmids. The numbers under each segment indicate distance in bp (map not drawn to scale). The numbers adjacent to each map are the sizes of the expected digestion products, with the asterisks indicating the product size that is unique to the particular configuration. ( b ) Digest analysis of loxP × loxP (left five lanes) and ψlox h7q21 × ψCore h7q21 (right five lanes) recombination. ( c , d ) Inversion and recombination frequency of ( c ) loxP × loxP and ( d ) ψlox h7q21 × ψCore h7q21 recombination obtained by quantifying band intensities. Error bars correspond to 95% CI ( n =two independent experiment). NI, Nco I site; SI, Sca I site. Full size image Achieving equilibrium in the inversion assay should result in 50% inversion. Recombination of two loxP sites by R32V, R32M and 303GVSdup resulted in ~50% inversion and no detectable deletion products. In contrast, WT resulted in deletion in 98.7% (95% confidence interval (CI): 97.5–100%) of plasmids ( Fig. 5c ). Unlike inversions, which can be reversed, excisions are selected for in a dividing cell population, because the excised products cannot replicate. Therefore, the data should not be taken to mean that WT incorrectly excises nearly 100% of the time, but rather that the vast majority of substrate plasmids experienced at least one excision event during the 12 h of growth. Recombination by WT of pseudo-loxP sites ψLox h7q21 and ψCore h7q21 resulted in improper excision with a frequency of 97.5% (95% CI: 96.5–98.4%). R32V, R32M and 303GVSdup produced no detectable recombination products ( Fig. 5d ). In aggregate, the data provided evidence that the isolated mutants are better able to distinguish on-target and off-target sites than WT. Mutants are functional in vitro and in human cells Given that in vivo recombination between two loxP sites reached equilibrium (~100% deletion for WT and ~50% inversion for R32V, R32M and 303GVSdup), there are two explanations for the improved selectivity against pseudo- loxP sites observed for the mutant recombinases; either the mutants were better able than WT to discriminate against pseudo- loxP sites or the mutants were equally less efficient at recombining loxP and pseudo- loxP sites than WT, but the high enzyme concentration and long reaction times were sufficient to drive loxP recombination to completion. These two hypotheses can be distinguished by comparing recombination of pseudo- loxP sites under conditions at which WT and mutants have comparable, subequilibrium efficiencies of loxP recombination. As such conditions can be easily found in vitro , we attempted to purify the WT and mutant Cre recombinases. Affinity purification of using a maltose-binding protein (MBP) domain fusion followed by scarless protease cleavage of at the MBP domain allowed isolation of WT, R32V and R32M ( Supplementary Fig. S2 ). We attribute our failure to purify 303GVSdup to its lack of solubility following MBP removal. We measured recombination kinetics using an intramolecular excision assay on linearized plasmid substrates. To test off-target activity, we used a pseudo- loxP site lox80 ( Fig. 3b ), which preliminary tests revealed to be efficiently recombined by WT in vitro . WT, R32V and R32M were all able to recombine loxP within the 8-h assay. In contrast to WT, R32V and R32M did not produce detectable loxP × lox80 reaction products ( Fig. 6a–c ). WT recombination of the loxP × lox80 substrate produced a small amount of an unexpected product that migrated at approximately twice the size of the linear recombination product. This product, which we excluded from our quantitative analysis, may represent recombination with a cryptic pseudo- loxP site in the vector backbone. 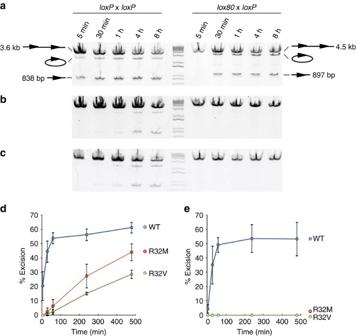Figure 6:In vitrorecombination of plasmids by mutants of Cre. (a) WT Cre purification ofloxP×loxP(left) andlox80×loxPsubstrates was performed for the indicated amount of time and resolved on an agarose gel. The linearized substrate plasmid contained two recombination sites such that catalysis resulted produced a circular and a short linear fragment. The same conditions were used to test (b) R32V and (c) R32M. The band intensities were quantified and plotted for (d)loxP×loxPand (e)lox80×loxPrecombination. Error bars correspond to 95% CI (n=two to four experiments using different protein preparations). Figure 6: In vitro recombination of plasmids by mutants of Cre. ( a ) WT Cre purification of loxP × loxP (left) and lox80 × loxP substrates was performed for the indicated amount of time and resolved on an agarose gel. The linearized substrate plasmid contained two recombination sites such that catalysis resulted produced a circular and a short linear fragment. The same conditions were used to test ( b ) R32V and ( c ) R32M. The band intensities were quantified and plotted for ( d ) loxP × loxP and ( e ) lox80 × loxP recombination. Error bars correspond to 95% CI ( n =two to four experiments using different protein preparations). Full size image Cre recombined loxP × loxP and lox80 × loxP reactions with comparable kinetics, although it was significantly less effective recombining lox80 at the 5-min time point ( Fig. 5d,e ). R32V and R32M recombined loxP sites significantly more slowly than WT, with both mutants failing to achieve a steady state within the 8-h experiment. The kinetic data enabled pseudo- loxP recombination efficiencies of the different mutants to be compared at similar loxP × loxP recombination efficiencies. For instance, after 5 min WT had recombined loxP sites with 21% efficiency, after 8 h R32V had recombined loxP sites with 29% efficiency and after 4 h R32M recombined the loxP substrate at an efficiency of 27%. Despite the slightly higher loxP recombination efficiencies, R43V and R32M had no detectable off-target activity, whereas WT recombined lox80 and loxP with 4% efficiency. A similar conclusion can be reached by comparing the 46% loxP × loxP efficiency and 35% lox80 × loxP achieved by WT after 30 min to the 44% loxP × loxP efficiency and absence of off-target recombination seen with R32M after 8 h. In aggregate, these data support the model under which the mutations we identified destabilize both loxP and pseudo- loxP recombination, but with a much greater reduction in pseudo- loxP efficiency than in loxP efficiency. Our observation that R32V and R32M are functional in vitro suggested that the mutants, such as Cre, could catalyse loxP recombination in mammals. To test the functionality of Cre mutants in human HEK293 cells, we expressed R32V, R32M and 303GVSdup under the control of the cytomegalovirus promoter. The substrate plasmid contained a loxP -flanked GFP with downstream lacZ gene, such that recombination excised GFP and made the cells turn blue when stained with X-gal ( Supplementary Fig. S3a ). Two and a half days following transfection with R32V, R32M and 303GVSdup, the cells had lost the GFP signal and stained positive for β-galactosidase activity ( Supplementary Fig. S3b ). As in E. coli , the in vivo reaction approached completion; the transfection efficiency-normalized recombination efficiencies were 95.2% for R32V (95% CI: 85.9–100%), 99% for R32M (95% CI: 97.1–100%) and 100% for 303GVSdup (with no variation across replicates; Supplementary Fig. S3c ). Mutants have less off-target activity genome wide One explanation for the improved accuracy we observed with R32V, R32M and 303GVSdup is that the mutations altered the preferred off-target sites without changing the overall accuracy. To test this possibility, we measured the efficiency of off-target insertions across the entire E. coli genome. Strains carrying the arabinose-inducible recombinase expression plasmids were transformed with a plasmid containing a loxP site, an R6k-γ origin of replication and a kanamycin resistance gene. As the R6k-γ origin cannot replicate in the pir− strain we used, only insertion of the plasmid into the genome would result in the replication of the kanamycin resistance gene. To control for variable transformation efficiencies, we normalized the number of R6k-γ colonies by the number of colonies arising from transformation with a plasmid lacking loxP but containing a functional origin of replication. We were unable to obtain Cre-mediated integration on LB/glucose. However, when we briefly pulsed the cells with arabinose before the growth on LB/glucose, we obtained a WT-mediated integration frequency of 1.3 × 10 −4 ( Table 1 ). 303GVSdup had an integration frequency ~100-fold lower than WT. The integration frequencies of R32V and R32M were lower than that of 303GVSdup and could not be distinguished from the Y324F background. These data strongly suggest that the higher accuracy of the mutants was not restricted to loxBait , ψLox h7q21 and lox80 . Table 1 Genome-wide off-target integration frequency. Full size table Our data suggest that R32V, R32M and 303GVSdup can efficiently recombine loxP in bacteria and in human cells. We also observed that the mutants exhibit better directionality and better accuracy with respect to the pseudo- loxP site ψLox h7q21 than WT Cre. R32V and R32M were functional in vitro and were better able to discriminate against the lox80 site than WT Cre. All three mutants more rarely integrated a loxP -carrying plasmid into the E. coli genome than WT Cre. Crystal structures of Cre strongly suggest that R32V and R32M disrupt a strong salt bridge in the dimer interface ( Fig. 4a ). The duplicated residues in the de novo 303GVSdup mutant are also located at the dimer interface, although the exact biochemical consequences of the mutation are unclear. Despite our model’s prediction that higher protein concentrations should reduce the accuracy of recombination ( Fig. 1 ), we saw identical results in our bacterial plasmid recombination assay when the P bad promoter controlling protein expression was repressed with glucose ( Fig. 5c,d ) and when it was weakly induced by LB without glucose. Despite the apparent contradiction, the data do not disprove the model. Even under glucose repression, WT Cre was able to drive both the loxP and pseudo- loxP reactions to equilibrium within the time frame of the experiment; therefore, any increases in recombination efficiency caused by a higher protein concentration could not be measured. The same logic applies to R32V, R32M and 303GVSdup recombining loxP sites. The model predicts that higher protein concentrations should cause Cre mutants to recombine pseudo- loxP sites more efficiently. The data neither confirm nor deny this prediction, as both expression conditions resulted in a recombination frequency that was below the detection level. The main limitation of our accuracy model is that it considers only binding, ignoring catalysis. The binding site sequence likely contributes to both establishing the proper alignment of the catalytic site and creating a tertiary DNA structure within the recombinase complex that is energetically favourable for recombination. The DNA site may also contribute to protein folding [35] . It is therefore possible that R32V, R32M and 303GVSdup mutations contribute to improved accuracy in steps of the catalytic pathway other than DNA binding. If that is the case, there may exist pseudo- loxP sites that are recombined by WT Cre but not at all by the mutants. Although R32V and R32M had high in vivo recombination efficiencies, the mutants catalysed recombination slower than WT in vitro ( Fig. 6d ). The slower kinetics may explain some of the decrease in apparent off-target integration in the genome-wide assay ( Table 1 ). However, during the genome integration assay, the cells were induced for 30 min and then recovered for 1 h in glucose media before antibiotic selection. If it is assumed that recombination occurred for 1 h (an underestimate, as recombination can continue to happen after the addition of antibiotics), then the in vitro data predict that R32V and R32M will produce 10- to 20-fold fewer transformants than WT. In fact, R32V and R32M were at least 200 times more accurate than WT. We therefore believe that the majority of the decrease in the frequency of genomic integration was caused by an improvement in selectivity against pseudo- loxP sites and not by the mutants’ slowed reaction kinetics. Our observation that Cre make frequent deletions on a substrate containing inverted loxP has been made previously [36] and is consistent with the fact that Cre can occasionally recombine sites with non-matching spacers [30] , [31] . This looseness in the directionality of recombination may interfere with synthetic circuit designs that rely on Cre-mediated inversion as a form of genetic memory [37] , [38] . The three Cre mutants we isolated seem to have an improved directionality over WT and may therefore be of use in synthetic biology applications. As the binding specificity of nucleases is the major determinant of their toxicity, it may be possible to minimize nucleases’ toxicity by reducing their DNA-binding cooperativity [39] . The main limitation of this approach is the fact that it inevitably decreases affinity for the target site. Strong monomer affinities, such as the 1–10 nM K d of Cre for half of loxP (refs 32 , 40 ), are a likely prerequisite. For comparison, DNA-binding domains composed of three Cys 2 –His 2 zinc fingers have been reported to bind to their 9 bp recognition sequence with a K d as low as 400 pM, whereas one 17.5 TALE repeat domain interacts with DNA with a K d of 160 pM (refs 41 , 42 ). Although only the better zinc finger and TALE designs achieve such high binding energies, the reported values suggest that destabilizing the cooperativity of DNA binding may be a viable strategy for increasing the accuracy of designer nucleases. Changing the dimer interface has been previously used to improve the specificity of nucleases engineered to cut asymmetrical DNA sites. As targeting asymmetric sites necessitates coexpression of two different DNA-binding domains fused to a constant nuclease domain, catalytically active dimers can form at four different sites: the desired asymmetric site, an off-target asymmetric site and the two symmetric sites targeted by the two possible homodimers. Converting the nuclease dimerization interface into a heterodimeric interface reduces activity at the two symmetric off-target sites [43] , [44] , [45] . The approach described in this paper is different from the obligate heterodimer strategy, because destabilizing the cooperativity of a dimeric protein improves accuracy by increasing the energy difference between binding to the target and the off-target sites—not by reducing the number of possible target sites. The obligate heterodimer and the destabilized cooperativity strategies should be compatible with each other, as it should be possible to modulate the binding cooperativity of heterodimers. Because of its high efficiency and the lack of necessary cofactors, Cre has found widespread use in genetics research [46] . However, Cre toxicity in the absence of loxP sites has been observed in a variety of animal and cell culture systems [47] , [48] , [49] , [50] , [51] . The source of this toxicity is not known. However, a number of observations, including the absence of toxicity from catalytically inactive Cre mutants, an increase in the frequency of chromosomal rearrangements and evidence of activation of DNA damage response pathways, all point at recombination at off-target pseudo- loxP sites as the cause [47] , [49] , [50] , [51] . We envision that the Cre mutants isolated in this study may be useful for alleviating the toxic phenotypes associated with WT Cre. This approach should be compatible with existing strategies for reducing Cre toxicity, which include placing the Cre gene in a self-excisable cassette, regulating Cre activity with a hormone-binding domain of a steroid receptor, or using a drug-regulated fragment complementation strategy [50] , [52] , [53] , [54] . Plasmid construction The positive selection substrate pCR-(loxP-ampR-loxP inv ) inv was built by amplifying ampR from pQL123 (ref. 55 ) with primers ampR_f and ampR_r (primer sequences are provided in Supplementary Table S1 ), performing an extension PCR on the amplicon with ampR_loxP_f and ampR_loxP_inv_r, and TOPO cloning the product into pCR-Blunt II-TOPO (Life Technologies). Sequencing was used to screen for colonies in which the ampR gene was in reverse orientation with respect to the promoter. A similar workflow was used to construct pCR-(h7q21-ampR-ψLox h7q21 inv ) inv , pCR-(lox80-ampR-loxP) inv and pCR-loxBait-ampR-loxP. The pZE2-loxP/loxP and pZE2-ψCore h7q21/ψLox h7q21 in vivo recombination substrates were obtained by cloning the Xho I/ Bam HI fragment from pCR-(loxP-ampR-loxP inv ) inv or pCR-(h7q21-ampR-ψLox h7q21 inv ) inv into Xho I/ Bam HI-digested pZE21G. The Cre gene was obtained from pQL123, although we reverted the alanine at the second position to the serine found in WT Cre (GenBank sequence YP_006472). For the bacterial assays, the Cre mutants or libraries were introduced in place of HpaII[51–358] in pARC8-HpaII[51–358] (a derivative of pAR-MHhaI[29–327] [56] containing residues 51–358 of Hpa II in the place of Hha I) using Gibson assembly [57] . Cloning was performed with a backbone amplified using primers pARC8_f and pARC8_r. For protein purification, WT, R32V, R32M and 303GVSdup were amplified from the respective pARC8-based plasmids using primers Cre_notATG_f and Cre_SalI_r. The genes were digested with Sal I and ligated into Sal I/ Xmn I-digested pMAL-c5x (New England Biolabs). For mammalian expression, R32V, R32M and 303GVSdup were amplified from the corresponding pARC8-based expression plasmids using primers Cre_TA_f and Cre_TA_r and TOPO TA cloned into pcDNA3.3-TOPO (Life Technologies). Clones were screened for the correct orientation by PCR. Identifying and characterizing functional loxP variants Libraries of half-site variants were constructed by amplifying the pZE21G plasmid [58] first with primers pZE21G_f and pZE21G_r, and then pZE21G_2_lib and pZE21G_2_loxP, producing an amplification product that was 2,437 bp long, and contained a loxP site and a random library site near each end. The libraries were purified using the QIAquick PCR Purification Kit (Qiagen), 10–20 ng of the DNA was treated with 1 U Cre (New England Biolabs) in Cre reaction buffer (10 mM MgCl 2 , 33 mM NaCl, 50 mM Tris-HCl pH 7.5) in 20 μl total reaction volume for 1 h at 37 °C, heat inactivated at 75–80 °C, then digested with Dpn I. The DNA was then purified, digested with PlasmidSafe (Epicentre) and transformed into One Shot Top10 chemically competent cells (Life Technologies; rec A1 ara D139 Δ( ara-leu )7697 Δ( lac )X74). Colonies were randomly selected for sequencing. Substrates for validating the selection hits were generated by performing extension PCR on pZE21G as for the selections, except that sequences obtained from the selection were in place of the random library. Thirty nanograms of purified products were treated with 1 U Cre in Cre reaction buffer, in 20 μl total reaction volume for 1.5 h at 37 °C, followed by heat inactivation of the enzyme. The entire reaction was resolved on a 0.7% agarose gel stained with SYBR Green I (Life Technologies). Each recombination was performed in parallel with a no-enzyme negative control. Negative and positive selections The pCR-(loxP-ampR-loxP inv ) inv and pCR-loxBait-ampR-loxP selection plasmids were maintained in NEB 10-beta cells (New England Biolabs; rec A1 ara D139 Δ( ara-leu )7697 Δ( lac )X74); cells were made electrocompetent using standard techniques [59] . The library of Cre variants was generated by mutagenic PCR using a pool of 19 oligonucleotides that substituted each of the 19 codons encoding S20–S38 for NNN (first round of PCR: primers Cre_mut_1—Cre_mut_19 and Cre_pARC8_r and second round of PCR: primers Cre_pARC8_f and Cre_pARC8_r). The library was introduced into pARC8 using Gibson assembly, desalted by drop dialysis and electroporated into competent cells carrying pCR-(loxP-ampR-loxP inv ) inv . Control transformations were performed with 100 pg pARC8-Cre or pARC8-Y324F. Transformed cells were recovered in low-salt 2 × LB (2% bacto-tryptone, 1% yeast extract, 0.5% NaCl, pH 7.5) at 37 °C for 30 min, induced with 0.2% arabinose at 37 °C for 30 min and recovered in SOC with 200 μM IPTG (isopropyl-β- D -thiogalactoside) at 37 °C for 1 h. The cells were then grown overnight at 37 °C on 0.2% glucose, 100 μM IPTG, 12.5 μg ml −1 chloramphenicol, 50 μg ml −1 kanamycin LB plates either with or without 100 μg ml −1 carbenicillin. Colonies obtained from the positive selection of the library and of the controls were collected by scraping. DNA was isolated using the QIAprep Spin Miniprep kit (Qiagen) and was digested with Xma I and Spe I (which cut only the substrate plasmids). The concentration of expression plasmid was quantified via agarose gels. Electrocompetent cells carrying the pCR-loxBait-ampR-loxP-negative selection substrate were transformed with 100 pg of the expression plasmid, recovered the cells in low-salt 2 × LB for at 28 °C for 30 min, induced with 0.2% arabinose at 28 °C for 30 min, washed with SOC and recovered in SOC with 200 μM IPTG at 37 °C for 1 h. The cells were then grown overnight at 37 °C on 0.2% glucose, 100 μM IPTG, 12.5 μg ml −1 chloramphenicol, 50 μg ml −1 kanamycin and 100 μg ml −1 carbenicillin LB plates. To ensure clonality, the isolated variants were amplified and re-cloned into pARC8 via Gibson assembly. Bacterial recombination assay Efficiencies were measured by cotransforming 75 ng of a pARC8-based expression plasmid (WT, Y324F, R32V, R32M or 303GVSdup) and an equimolar amount of either pZE2-loxP/loxP or pZE2-ψCore h7q21/ ψlox h7q21 into 50 μl vial of One Shot Top10 chemically competent cells. The cells were recovered in LB with 0.2% glucose at 37 °C for 1 h, then grown at 37 °C for 12 h in 0.2% glucose, 12.5 μg ml −1 chloramphenicol and 50 μg ml −1 kanamycin LB. The plasmids were isolated using the QIAprep Spin Miniprep kit, eluting into 50 μl of 10 mM Tris-HCl pH 8. The purified plasmids were digested for 20 min at 37 °C in 60-μl reactions containing all of the collected DNA and 20 U of both Sca I-HF and Nco I-HF (both from New England Biolabs) in NEBuffer 4 (1 mM dithiothreitol (DTT), 50 mM potassium acetate, 20 mM tris-acetate, 10 mM magnesium acetate, pH 7.9). The digests quantified on 1% agarose gels following purification using the QIAprep Spin Miniprep kit. In vitro recombination assay The pMAL-based recombinase expression plasmids were maintained in One Shot Top10 chemically competent cells. An overnight culture of each expression clone was diluted to OD 600 of 0.02 in 55 ml 0.2% glucose, 50 μg ml −1 kanamycin LB and grown for 2.5 h at 37 °C. IPTG was added to a final concentration of 300 μM and the cultures were grown at 37 °C for an additional 2 h. Fifty millilitres of the culture were pelleted, resuspended in 5 ml lysis buffer (1 mM EDTA, 1 mM DTT, 200 mM NaCl, 20 mM Tris-HCl pH 8) supplemented with Halt Protease Inhibitor Cocktail (Thermo Scientific). The cell suspension was lysed using eight 15 s sonication cycles using a power setting of 4 on a Misonix Sonicator 3000. The lysate was centrifuged for 20 min at 5,000 g and the supernate was bound to 500 μl amylose resin (New England Biolabs). The resin was washed with 4 ml wash buffer (200 mM NaCl, 20 Tris-HCl pH 7.5), 12 ml of DNA-removal buffer (1 M NaCl, 20 mM Tris-HCl pH 7.5) and again with 4 ml wash buffer. The protein was eluted into 500 μl elution buffer (0.5% maltose, 2 mM CaCl 2 , 100 mM NaCl, 20 mM Tris-HCl pH 7.5) and digested with 200 ng Factor Xa (New England Biolabs) for 13–14 h at room temperature. The protease activity was stopped by adding 1 × Halt Protease Inhibitors and 1 mM DTT. Precipitated protein was removed by centrifuging at 16,000 g for 10 min and passing the supernate through an Amicon Ultracel 100K filter. The flowthrough was concentrated using an Amicon Ultracel 10K filter. Glycerol was added to 27% final volume, NaCl was added to adjust the concentration to 200 mM and the proteins were stored at −20 °C. Catalytic assays were performed within 2 days of purification. Protein concentration was determined using a Qubit 2.0 fluorometer (Life Technologies). The concentration of protease-cleaved recombinase was determined by quantifying band intensity on a SimplyBlue (Life Technologies)-stained PAGE gel (typical values were 15–30%) and then by normalizing the total protein concentration by the obtained value. Linearized pLox2+ (New England Biolabs) and Sca I-digested pCR-(lox80-ampR-loxP) inv were used as the recombination substrates. Recombination kinetics were measured by reacting 5 nM of the DNA substrate and 750 nM of each protease-cleaved recombinase in Cre reaction buffer with 100 ng μl −1 BSA. The reactions were performed at 37 °C and were stopped by heating them to 70 °C for 15–25 min. Excision was measured by quantifying bands on 1% agarose gels. Human cell culture recombination assay pCMV:GFP(loxP)lacZ (ref. 60 ; Addgene: 31125) was used as the recombination substrate plasmid and pcDNA3.3-TOPO/lacZ (Life Technologies) was used as a lacZ staining control. Except for pcDNA3.3-TOPO/lacZ, which was prepared by the manufacturer, all substrate and expression plasmids were prepared for transfection using the HiSpeed Plasmid Maxi Kit (Qiagen). Lenti-X 293T cells (Clontech) were grown on poly- D -lysine–coated, tissue-culture-treated polystyrine in DMEM High Glucose with GlutaMAX (Life Technologies) supplemented with 10% fetal bovines serum, 50 U ml −1 penicillin and 50 μg ml −1 streptomycin at 37 °C and 5% CO 2 in a humidified incubator. Cells were subcultured using TrypLE Express (Life Technologies). Cells in 12-well plates were transformed with 500 ng pCMV:GFP(loxP)lacZ and 500 ng pcDNA3.3-TOPO-based expression plasmid using Fugene HD (Promega). Substrate-only controls were transformed with 500 ng recombination substrate and the lacZ controls were trasfromed with 500 ng pcDNA3.3-TOPO/lacZ. Media was changed 1 day following transfection. Cells were subcultured 2 days following transfection. Staining and imaging was performed 2.5 days following transfection. Cells were fixed using 2% formaldehyde and 0.1% glutaraldehyde in PBS for 10 min at room temperature. After being washed with PBS, the cells were stained with 1 mg ml −1 X-gal, 4 mM potassium ferricyanide, 4 mM potassium ferrocyanide and 2 mM MgCl 2 in PBS for 30 min at 37 °C. Following staining, the cells were washed with PBS and imaged. Genome-wide off-target integration assay Electrocompetent cells were prepared from each of the pARC8-based expression plasmids (WT, Y324F, R32V, R32M or 303GVSdup) cloned in NEB 10-beta cells using 40 ml of culture per transformation. Each expression strain was transformed either with 200 ng pUNI10 (loxP + , ori R6Kγ and kanR) (ref. 55 ) or an equimolar amount of pZE21G (loxP − , ori ColE1 and kanR). The two transformations were done in parallel using competent cells made from aliquots of the same culture. The cells were recovered in LB for at 37 °C for 30 min, induced with 0.2% arabinose at 37 °C for 30 min and recovered in SOC at 37 °C for 1 h. The cells were then grown overnight at 37 °C on 0.2% glucose, 12.5 μg ml −1 chloramphenicol and 50 μg ml −1 kanamycin LB plates. How to cite this article: Eroshenko, N. and George, M.C. Mutants of Cre recombinase with improved accuracy. Nat. Commun. 4:2509 doi: 10.1038/ncomms3509 (2013)